FBXW7α attenuates inflammatory signalling by downregulating C/EBPδ and its target geneTlr4 Toll-like receptor 4 (Tlr4) has a pivotal role in innate immune responses, and the transcription factor CCAAT/enhancer binding protein delta (C/EBPδ, Cebpd ) is a Tlr4-induced gene. Here we identify a positive feedback loop in which C/EBPδ activates Tlr4 gene expression in macrophages and tumour cells. In addition, we discovered a negative feedback loop whereby the tumour suppressor FBXW7α (FBW7, Cdc4), whose gene expression is inhibited by C/EBPδ, targets C/EBPδ for degradation when C/EBPδ is phosphorylated by GSK-3β. Consequently, FBXW7α suppresses Tlr4 expression and responses to the ligand lipopolysaccharide. FBXW7α depletion alone is sufficient to augment pro-inflammatory signalling in vivo . Moreover, as inflammatory pathways are known to modulate tumour biology, Cebpd null mammary tumours, which have reduced metastatic potential, show altered expression of inflammation-associated genes. Together, these findings reveal a role for C/EBPδ upstream of Tlr4 signalling and uncover a function for FBXW7α as an attenuator of inflammatory signalling. Innate immune responses to infection are induced in part by Toll-like receptors (TLRs), which belong to the pattern recognition receptor family. To date, 10 human and 12 mouse TLRs are known, each of which binds specific ligands. TLR4 recognizes lipopolysaccharide (LPS) from Gram-negative bacteria and signals in combination with other co-receptors to activate the NF-kB transcription factors [1] . TLR4 is involved in diseases such as sepsis and chronic inflammatory disorders [2] , [3] . TLR4 signalling in tumour cells is associated with suppression of immune surveillance, proliferation, inflammatory cytokine production and invasive migration [4] , [5] , [6] , [7] , [8] . Therefore, understanding the regulation of TLR4 expression and signalling may be important for the management of these conditions. C/EBPδ is an inflammatory response gene [9] . C/EBPδ amplifies LPS signalling, and it is essential for the expression of many LPS-induced genes and the clearance of Gram-negative bacterial infection [10] . Cebpd deficiency partly protects mice from LPS-induced mortality and autoimmune encephalomyelitis, suggesting that C/EBPδ has a role in the progression of systemic inflammatory diseases such as sepsis and multiple sclerosis [11] , [12] . We reported that C/EBPδ directly inhibits the expression of the F-box and WD repeat domain containing protein 7 alpha (FBXW7α) in mammary tumour cells [13] . The Fbxw7 gene encodes three protein isoforms, of which the alpha isoform is the most abundantly expressed [14] . FBXW7 functions as the substrate-recognition subunit of SCF-type ubiquitin ligase complexes. FBXW7α targets various mammalian oncoproteins for degradation, including c-myc, cyclin E, mTOR, c-jun and Notch [14] , [15] . We also showed that hypoxia-induced C/EBPδ inhibited the expression of FBXW7α, resulting in elevated levels of mTOR and consequently hypoxia-inducible factor 1 alpha (HIF-1α) [13] . HIF-1α is a subunit of the HIF-1 transcription factor complex and is necessary for cellular adaptation to hypoxia. HIF-1 target genes promote angiogenesis and the metabolic switch to glycolysis, which augments survival under hypoxia [16] . In agreement with the role of hypoxia and HIF-1α in tumour metastasis [17] , [18] , loss of Cebpd results in reduced metastatic progression of MMTV-Neu-induced mammary tumours [13] . MMTV-Neu transgenic mice express the rat tyrosine kinase receptor Neu (ERBB2/HER2) specifically in mammary epithelial cells, mimicking the overexpression of ERBB2 observed in 30% of human breast cancers [19] . Although Cebpd -deficient MMTV-Neu-transgenic mice are 50% less likely than wild-type mice to develop metastases, these mice also exhibit a 50% increased tumour multiplicity compared with controls [13] ; this observation is in agreement with other tumour-suppressor like activities of C/EBPδ, such as suppression of cyclin D1 expression [13] , [20] , [21] . HIF-1α also promotes macrophage activation and inflammatory responses, as does the FBXW7α target Notch [22] , [23] . However, the role of FBXW7α in inflammatory signalling has not been addressed. As C/EBPδ augments HIF-1α expression in tumour cells [13] , and both C/EBPδ and HIF-1α are known to mediate inflammatory responses, we hypothesized that the C/EBPδ-FBXW7-HIF-1 pathway had a role in macrophage activation. Here, we show that C/EBPδ augments HIF-1α expression and pro-inflammatory signalling in activated macrophages through the inhibition of FBXW7α expression. We also found that C/EBPδ acts upstream of LPS signalling by directly activating Tlr4 gene expression. In addition, we identified a negative feedback loop where FBXW7α downregulates C/EBPδ that is phosphorylated by GSK-3β. These results identify a novel role for FBXW7α as a suppressor of inflammatory gene expression. LPS and C/EBPδ inhibit FBXW7α expression in macrophages We previously reported that C/EBPδ directly inhibits Fbxw7α gene expression in tumour cells, which in turn augments HIF-1α expression [13] . To investigate this pathway in macrophages, we first analysed FBXW7 isoform expression. Semi-quantitative analysis suggested that macrophages and mammary tumours expressed only Fbxw7α mRNA but not Fbxw7β or Fbxw7γ , while all three isoforms were detected in mouse embryo fibroblasts ( Fig. 1a ). In mouse primary peritoneal macrophages (PPMs), basal levels of Fbxw7α mRNA were higher in Cebpd −/− (KO) compared with wild-type (WT) macrophages. LPS treatment decreased Fbxw7α transcripts in WT but not in KO macrophages ( Fig. 1b ). The silencing of CEBPD by RNA interference (RNAi) in U-937 human monocytic cells increased the basal level of FBXW7 mRNA and abolished its repression upon LPS treatment ( Supplementary Fig. S1a ). Next, we analysed resident peritoneal exudate cells (PECs), which consisted of ~67±2.7% macrophages/monocytes, 23±1% lymphoid cells and 4.9±0.6% neutrophils independent of genotype (mean±s.e.m, n =4 mice). In vivo LPS treatment (6 h) reduced FBXW7α protein levels in WT PECs but not in Cebpd −/− cells, while C/EBPδ expression was induced by this treatment in WT PECs ( Supplementary Fig. S1b ). Furthermore, the higher levels of basal FBXW7α that were observed in Cebpd −/− PECs ( Supplementary Fig. S1b, c ) were correlated with reduced levels of its targets mTOR and Aurora A and reduced phosphorylation of AKT, S6K1 and GSK-3β ( Supplementary Fig. S1c ). Taken together, these data show that macrophages express FBXW7α and that FBXW7α expression is downregulated by C/EBPδ and LPS. 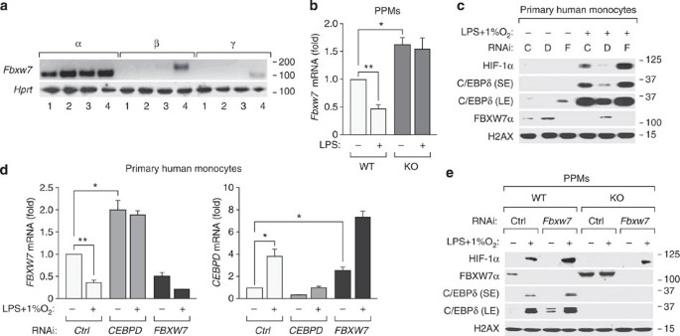Figure 1: C/EBPδ promotes HIF-1α expression in macrophages through inhibition of FBXW7α. (a) RT–PCR analysis of FBXW7 isoform expression from different sources as follows. (1) primary peritoneal macrophages (PPMs); (2) RAW 264.7 cells; (3) MMTV-Neu mammary tumour tissue; (4) primary mouse embryo fibroblasts. Numbers indicate the position of size markers in base pairs. (b) RT–qPCR analysis ofFbxw7transcript levels in PPMs from WT andCebpd−/−mice, cultured +/− LPS (100 ng ml−1, 24 h), compared with WT untreated (n=4, *P<0.05; **P<0.001). (c) Western analysis of nuclear extract (NE) from primary human monocytes nucleofected with siRNA oligos (C, control; D, CEBPD;F, FBXW7) and treated with LPS (100 ng ml−1) and 1%O2(16 h) as indicated. SE, short exposure; LE, long exposure. (d) RT–qPCR analysis ofFBXW7andCEBPDtranscripts in primary human monocytes as in panel (c) (n=3, *P<0.05; **P<0.001). (e) Western analysis of NE from PPMs nucelofected with siRNA oligos and treated with LPS (100 ng ml−1) and 1% O2for 16 h as indicated. SE, short exposure; LE, long exposure. Where applicable, data are mean±s.e.m., evaluated by two-tailed unequal variancet-test. Figure 1: C/EBPδ promotes HIF-1α expression in macrophages through inhibition of FBXW7α. ( a ) RT–PCR analysis of FBXW7 isoform expression from different sources as follows. (1) primary peritoneal macrophages (PPMs); (2) RAW 264.7 cells; (3) MMTV-Neu mammary tumour tissue; (4) primary mouse embryo fibroblasts. Numbers indicate the position of size markers in base pairs. ( b ) RT–qPCR analysis of Fbxw7 transcript levels in PPMs from WT and Cebpd −/− mice, cultured +/− LPS (100 ng ml −1 , 24 h), compared with WT untreated ( n =4, * P <0.05; ** P <0.001). ( c ) Western analysis of nuclear extract (NE) from primary human monocytes nucleofected with siRNA oligos (C, control; D , CEBPD; F , FBXW7 ) and treated with LPS (100 ng ml −1 ) and 1%O 2 (16 h) as indicated. SE, short exposure; LE, long exposure. ( d ) RT–qPCR analysis of FBXW7 and CEBPD transcripts in primary human monocytes as in panel ( c ) ( n =3, * P <0.05; ** P <0.001). ( e ) Western analysis of NE from PPMs nucelofected with siRNA oligos and treated with LPS (100 ng ml −1 ) and 1% O 2 for 16 h as indicated. SE, short exposure; LE, long exposure. Where applicable, data are mean±s.e.m., evaluated by two-tailed unequal variance t -test. Full size image C/EBPδ and FBXW7α control HIF-1α expression in monocytes LPS and hypoxia cooperatively induce HIF-1α expression in macrophages [24] , and we confirmed these results in ANA-1 mouse macrophages ( Supplementary Fig. S1d ). Under these conditions, primary human monocytes treated with CEBPD RNAi had increased FBXW7α expression and reduced HIF-1α accumulation ( Fig. 1c ). As expected [13] , CEBPD depletion also increased FBXW7α mRNA levels ( Fig. 1d ). Interestingly, FBXW7α depletion increased the levels of C/EBPδ and HIF-1α protein ( Fig. 1c ) and of CEBPD mRNA ( Fig. 1d ), demonstrating that FBXW7α suppresses C/EBPδ expression. In Cebpd −/− PPMs, HIF-1α accumulation could be rescued by knockdown of the elevated FBXW7α ( Fig. 1e ). These results demonstrate that C/EBPδ promotes HIF-1α expression in activated macrophages through the inhibition of FBXW7α expression, as previously reported for mammary tumour cells [13] . HIF-1 is critical for hypoxia-induced glycolysis in macrophages [22] . Therefore, we examined if reduced HIF-1α expression in Cebpd null PECs affected their glycolytic activity and activation. Under inflammatory conditions (LPS+1% O 2 ), Cebpd null PECs exhibited reduced hallmarks of the glycolytic switch, such as glucose consumption and lactate generation ( Supplementary Fig. S1e ). In agreement with these data, ATP production and the survival of Cebpd null peritoneal cells were reduced under these conditions ( Supplementary Fig. S1f-g ). Furthermore, Cebpd -deficient peritoneal macrophages exhibited limited induction of pro-inflammatory genes, such as Mmp9 , Cxcr4 , Vegfc and Il6 , after stimulation with LPS+1% O 2 ( Supplementary Fig. S1h ). These genes are known HIF-1 targets [18] ; Il6 and Cxcr4 are also direct targets of C/EBPδ [10] , [13] . Collectively, these findings show that C/EBPδ supports HIF-1-mediated inflammatory responses. Importantly, there was no difference in the number of PECs isolated from Cebpd −/− mice compared with the controls. However, there was a small but significant decrease in the number of PPMs isolated from Cebpd −/− mice after elicitation, and there was a significant decrease in the recruitment of peritoneal cells upon LPS treatment in vivo ( Supplementary Fig. S2a,b ). An analysis of baseline myeloid haematopoiesis suggests that myeloid development is normal in Cebpd −/− mice (see Supplementary Note 1 and Supplementary Fig. S2c-j ). Thus, we conclude that the functional differences detected in the macrophages from Cebpd −/− mice are not due to developmental defects. FBXW7α targets C/EBPδ for degradation FBXW7α is not a transcription factor. Therefore, its downregulation of Cebpd mRNA levels must be through indirect mechanisms. As C/EBPδ can activate its own promoter [10] and has a degron-like sequence commonly found in FBXW7 substrates [14] , [15] , we investigated whether FBXW7α regulated C/EBPδ expression at the protein level. Pulse-chase analysis ( Fig. 2a ) and cycloheximide-chase experiments ( Supplementary Fig. S3a ) showed that the half-life of C/EBPδ protein increased significantly when Fbxw7α was silenced in RAW 264.7 macrophages. Furthermore, inhibition of the proteasome by MG132 increased the basal expression of C/EBPδ and revealed its polyubiquitination, which was significantly reduced upon Fbxw7α silencing ( Fig. 2b and Supplementary Fig. S3b ). In Fbxw7α -silenced cells, MG132 did not further increase C/EBPδ protein levels. In contrast, ectopic FBXW7α [25] further decreased the half-life of C/EBPδ and increased its polyubiquitination ( Supplementary Fig. S3c,d ). Co-immunoprecipitation assays showed that ectopic and endogenous C/EBPδ physically interacted with FBXW7α ( Supplementary Fig. S3e ). These results indicate that FBXW7α is required for the ubiquitination and degradation of C/EBPδ in RAW 264.7 macrophages. Accordingly, C/EBPδ binding to its own promoter increased when Fbxw7α was silenced ( Supplementary Fig. S3f ). Collectively, these data demonstrate a negative feedback loop from FBXW7α to C/EBPδ. 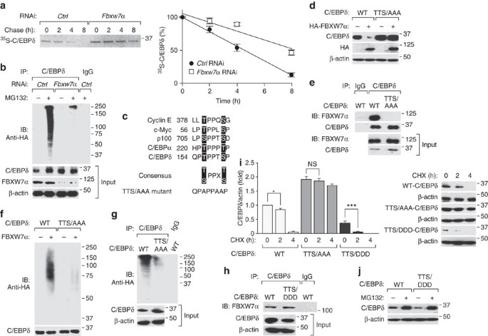Figure 2: FBXW7α interacts with C/EBPδ and targets it for degradation. (a) RAW 264.7 macrophages were transfected with control orFbxw7αsiRNA oligos for 48 h, then pulse-labelled with35S-methionine/cysteine, followed by chased with excess unlabelled aminoacids for the indicated times. Quantitation of the phosphorimage of C/EBPδ signal is depicted in the graph (mean±s.e.m.,n=2–3) and representative primary data are shown. (b) Western analysis of RAW 264.7 cells transfected with HA-ubiquitin expression constructs and control orFbxw7αsiRNA oligos and treated ± MG132 (20 μM, 6 h), followed by immunoprecipitation under denatured conditions with anti-C/EBPδ or IgG (with equal aliquots of the indicated extracts). Input (2.5% of lysate) was analysed as indicated. (c) Alignment of phosphodegron motifs present in known FBXW7 substrates with C/EBPδ and its TTS/AAA mutant. (d) Western analysis of RAW 264.7 cells transfected with WT- or TTS/AAA-CEBPδ expression plasmids and/or HA-FBXW7α. (e) Western analysis of RAW 264.7 cells transfected with W-T or TTS/AAA-C/EBPδ expression plasmids and immunoprecipitated with anti-C/EBPδ or IgG and input (2.5% of lysate) as indicated. (f) RAW 264.7 cells were transfected with WT- or TTS/AAA-C/EBPδ expression constructs. C/EBPδ was immunoprecipitated and the beads were incubated with FBXW7α and HA-ubiquitin as indicated (see Methods for details) and analysed by western with anti-HA and C/EBPδ antibodies. (g) Western analysis of RAW 264.7 cells transfected with WT- or TTS/AAA-C/EBPδ, treated ± MG132 (20 μM, 6 h) followed by immunoprecipitation under denatured conditions using anti-C/EBPδ or IgG and input (2.5% of lysate) as indicated. (h) Western analysis of RAW 264.7 cells transfected with WT- and TTS/DDD-C/EBPδ for 48 h followed by immunoprecipitation with anti-C/EBPδ or IgG and input (2.5% of lysate) as indicated. (i) Western analysis (right panel) of RAW 264.7 cells transfected with WT-, TTS/AAA- or TTS/DDD-C/EBPδ expression constructs and treated with CHX as indicated. Quantification (left panel) of the C/EBPδ signal was normalized to actin (n=3, *P<0.05; ***P<0.0001; NS, not significant). (j) Western analysis of RAW 264.7 cells transfected with WT- or TTS/DDD-C/EBPδ expression constructs and treated ±MG132 (20 μM, 6 h). Where applicable, data are mean±s.e.m., evaluated by two-tailed unequal variancet-test. Figure 2: FBXW7α interacts with C/EBPδ and targets it for degradation. ( a ) RAW 264.7 macrophages were transfected with control or Fbxw7α siRNA oligos for 48 h, then pulse-labelled with 35 S-methionine/cysteine, followed by chased with excess unlabelled aminoacids for the indicated times. Quantitation of the phosphorimage of C/EBPδ signal is depicted in the graph (mean±s.e.m., n =2–3) and representative primary data are shown. ( b ) Western analysis of RAW 264.7 cells transfected with HA-ubiquitin expression constructs and control or Fbxw7α siRNA oligos and treated ± MG132 (20 μM, 6 h), followed by immunoprecipitation under denatured conditions with anti-C/EBPδ or IgG (with equal aliquots of the indicated extracts). Input (2.5% of lysate) was analysed as indicated. ( c ) Alignment of phosphodegron motifs present in known FBXW7 substrates with C/EBPδ and its TTS/AAA mutant. ( d ) Western analysis of RAW 264.7 cells transfected with WT- or TTS/AAA-CEBPδ expression plasmids and/or HA-FBXW7α. ( e ) Western analysis of RAW 264.7 cells transfected with W-T or TTS/AAA-C/EBPδ expression plasmids and immunoprecipitated with anti-C/EBPδ or IgG and input (2.5% of lysate) as indicated. ( f ) RAW 264.7 cells were transfected with WT- or TTS/AAA-C/EBPδ expression constructs. C/EBPδ was immunoprecipitated and the beads were incubated with FBXW7α and HA-ubiquitin as indicated (see Methods for details) and analysed by western with anti-HA and C/EBPδ antibodies. ( g ) Western analysis of RAW 264.7 cells transfected with WT- or TTS/AAA-C/EBPδ, treated ± MG132 (20 μM, 6 h) followed by immunoprecipitation under denatured conditions using anti-C/EBPδ or IgG and input (2.5% of lysate) as indicated. ( h ) Western analysis of RAW 264.7 cells transfected with WT- and TTS/DDD-C/EBPδ for 48 h followed by immunoprecipitation with anti-C/EBPδ or IgG and input (2.5% of lysate) as indicated. (i) Western analysis (right panel) of RAW 264.7 cells transfected with WT-, TTS/AAA- or TTS/DDD-C/EBPδ expression constructs and treated with CHX as indicated. Quantification (left panel) of the C/EBPδ signal was normalized to actin ( n =3, * P <0.05; *** P <0.0001; NS, not significant). ( j ) Western analysis of RAW 264.7 cells transfected with WT- or TTS/DDD-C/EBPδ expression constructs and treated ±MG132 (20 μM, 6 h). Where applicable, data are mean±s.e.m., evaluated by two-tailed unequal variance t -test. Full size image FBXW7-substrate interaction requires a phospho-degron motif, which is also present in C/EBPδ ( Fig. 2c ). To investigate the role of this motif, we mutated the potential phospho-acceptor residues serine and threonine to alanine (TTS/AAA). Figure 2d shows that FBXW7α decreased the steady-state levels of the ectopic wild-type C/EBPδ but not the TTS/AAA mutant. Co-immunoprecipitation assays revealed that the degron motif of C/EBPδ was necessary for its interaction with FBXW7α ( Fig. 2e ). Indeed, FBXW7α mediated the polyubiquitination of WT- but not TTS/AAA-C/EBPδ in vitro ( Fig. 2f ), and the degron motif was required for polyubiquitination in vivo ( Fig. 2g ). Next, we generated a TTS/DDD mutation to mimic its phosphorylation, and we confirmed that this protein interacted with FBXW7α ( Fig. 2h ). The half-life of TTS/DDD-C/EBPδ was significantly reduced compared with the stabilization observed with the TTS/AAA mutation ( Fig. 2i ). In the presence of MG132, WT- and TTS/DDD-C/EBPδ were expressed at similar steady-state levels; these findings corroborated the notion that the low levels of TTS/DDD-C/EBPδ were due to degradation ( Fig. 2j ). Collectively, these data show that degron-phosphorylation regulates the stability of C/EBPδ. GSK-3β regulates C/EBPδ protein stability The serine/threonine kinase GSK-3β is responsible for the phosphorylation of most FBXW7α substrates [14] . Indeed, phospho-threonine could be detected on WT-C/EBPδ expressed in RAW 264.7 cells, but this phosphorylation was significantly reduced by the GSK-3β inhibitor CHIR or the TTS/AAA mutation ( Fig. 3a ). Consistent with this result, the GSK-3β inhibitors CHIR or BIO increased the expression of C/EBPδ in PPMs and RAW 264.7 cells ( Fig. 3b ). In contrast, the expression of TTS/DDD-C/EBPδ was not increased by CHIR ( Fig. 3c ). These results suggest a role for the GSK-3β pathway in the regulation of C/EBPδ expression. Indeed, in vitro kinase assays with recombinant activated GSK-3β confirmed that GSK-3β directly phosphorylated C/EBPδ ( Fig. 3d ). The TTS/AAA mutation significantly reduced C/EBPδ phosphorylation, and phospho-peptide analysis confirmed that GSK-3β targets T156 of the degron ( Fig. 3d and Table 1 ). Phosphorylation at S160 was also detected but to a much lesser extent. In addition, T49 was phosphorylated by GSK-3β in vitro on both WT- and TTS/AAA-C/EBPδ. This residue is not conserved across species and its role, if any, remains to be determined. 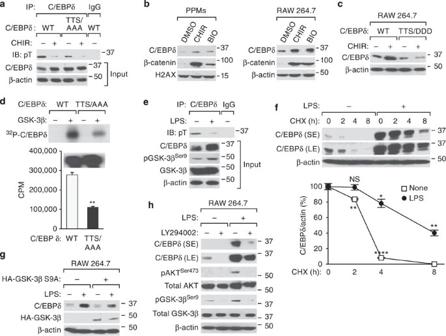Figure 3: C/EBPδ stability is regulated by GSK-3β phosphorylation. (a) RAW 264.7 cells were transfected with WT- or TTS/AAA-CEBPδ expression plasmids and treated ± GSK-3β inhibitor CHIR99021 (5 μM, 2 h). Cell extracts were immunoprecipitated with anti-C/EBPδ or IgG (with an aliquot of the indicated extract) and the western analysed with anti-phosphothreonine (pT) antibody. (b) Western analysis of NE from PPMs (left panel) or RAW 264.7 cells (right panel) treated with GSK-3β inhibitors CHIR99021 or BIO (6-bromoindirubin-3′-oxime) (5 μM, 2 h). β-catenin, which is known to be targeted for degradation by GSK-3β phosphorylation, served as positive control. (c) Western analysis of RAW 264.7 cells transfected with WT- or TTS/DDD-C/EBPδ expression plasmids and treated ± GSK-3β inhibitor CHIR99021 for 2 h. (d) GSK-3β phosphorylates C/EBPδin vitro. HEK293T cells were transfected with WT- or TTS/AAA-C/EBPδ expression plasmids. C/EBPδ proteins were immunoprecipitated from cell extracts andin vitrokinase assay reactions were carried out in the presence or absence of GSK-3β. Samples were resolved by SDS–PAGE and subjected to autoradiography (top panel). Total radioactivity (bottom panel) incorporated into the C/EBPδ protein was quantified (n=3). Representative input levels of C/EBPδ are shown by western (inset). (e) RAW 264.7 cells were treated ± LPS (4 h) and cell extracts were immunoprecipitated with anti-C/EBPδ or IgG antibodies and western analysis was carried out with anti-phosphothreonine (pT) antibody. Input (2.5% of the lysate) was analysed as indicated. (f) Western analysis (top panel) of RAW 264.7 cells treated ± LPS (100 ng ml−1, 4 h) followed by CHX for the indicated times, and quantification of C/EBPδ normalized to β-actin signal (bottom graph) compared with respective untreated (n=3, *P<0.05; **P<0.001; ****P<0.0001). (g) Western analysis of RAW 264.7 cells transfected with HA-GSK-3β-S9A expression plasmids treated ± LPS (4 h) as indicated. (h) Western analysis of RAW 264.7 cells pretreated with the PI3K/AKT kinase pathway inhibitor LY294002 (10 μM, 1 h) followed by LPS (100 ng ml−1, 4 h) as indicated. Where applicable, data are mean±s.e.m., evaluated by two-tailed unequal variancet-test. Figure 3: C/EBPδ stability is regulated by GSK-3β phosphorylation. ( a ) RAW 264.7 cells were transfected with WT- or TTS/AAA-CEBPδ expression plasmids and treated ± GSK-3β inhibitor CHIR99021 (5 μM, 2 h). Cell extracts were immunoprecipitated with anti-C/EBPδ or IgG (with an aliquot of the indicated extract) and the western analysed with anti-phosphothreonine (pT) antibody. ( b ) Western analysis of NE from PPMs (left panel) or RAW 264.7 cells (right panel) treated with GSK-3β inhibitors CHIR99021 or BIO (6-bromoindirubin-3′-oxime) (5 μM, 2 h). β-catenin, which is known to be targeted for degradation by GSK-3β phosphorylation, served as positive control. ( c ) Western analysis of RAW 264.7 cells transfected with WT- or TTS/DDD-C/EBPδ expression plasmids and treated ± GSK-3β inhibitor CHIR99021 for 2 h. ( d ) GSK-3β phosphorylates C/EBPδ in vitro . HEK293T cells were transfected with WT- or TTS/AAA-C/EBPδ expression plasmids. C/EBPδ proteins were immunoprecipitated from cell extracts and in vitro kinase assay reactions were carried out in the presence or absence of GSK-3β. Samples were resolved by SDS–PAGE and subjected to autoradiography (top panel). Total radioactivity (bottom panel) incorporated into the C/EBPδ protein was quantified ( n =3). Representative input levels of C/EBPδ are shown by western (inset). ( e ) RAW 264.7 cells were treated ± LPS (4 h) and cell extracts were immunoprecipitated with anti-C/EBPδ or IgG antibodies and western analysis was carried out with anti-phosphothreonine (pT) antibody. Input (2.5% of the lysate) was analysed as indicated. ( f ) Western analysis (top panel) of RAW 264.7 cells treated ± LPS (100 ng ml −1 , 4 h) followed by CHX for the indicated times, and quantification of C/EBPδ normalized to β-actin signal (bottom graph) compared with respective untreated ( n =3, * P <0.05; ** P <0.001; **** P <0.0001). ( g ) Western analysis of RAW 264.7 cells transfected with HA-GSK-3β-S9A expression plasmids treated ± LPS (4 h) as indicated. ( h ) Western analysis of RAW 264.7 cells pretreated with the PI3K/AKT kinase pathway inhibitor LY294002 (10 μM, 1 h) followed by LPS (100 ng ml −1 , 4 h) as indicated. Where applicable, data are mean±s.e.m., evaluated by two-tailed unequal variance t -test. Full size image Table 1 Sites of C/EBPδ phosphorylated by GSK-3β. Full size table Our results show that GSK-3β phosphorylation attenuates C/EBPδ levels in untreated macrophages. Next, we investigated the role of this pathway in activated macrophages. LPS signalling inhibits GSK-3β through the PI3K/AKT pathway [26] . LPS reduced threonine-phosphorylation of C/EBPδ, which was consistent with an increase in the inhibitory Ser9-phosphorylation on GSK-3β ( Fig. 3e ) and in the half-life of C/EBPδ ( Fig. 3f ). Furthermore, ectopic active GSK-3β-S9A [27] ( Fig. 3g ) or pharmacological inhibition of PI3K/AKT ( Fig. 3h ) reduced LPS-induced C/EBPδ expression. These data show that LPS activates C/EBPδ expression at least in part by inhibition of the GSK-3β/FBXW7α pathway. FBXW7α regulates TLR4 expression through C/EBPδ As FBXW7α targeted C/EBPδ for degradation, FBXW7α could have a role in attenuating pro-inflammatory signalling. To test this hypothesis, we expressed FBXW7α [25] in PPMs to mimic the elevated levels of FBXW7α in Cebpd null cells ( Supplementary Fig. S4a ). FBXW7α suppressed all tested responses of PPMs to LPS, such as the expression of iNOS, C/EBPδ, p65, Notch-intracellular-domain (NICD) and COX-2 and the phosphorylation of ERK1/2 and STAT3 ( Fig. 4a ). Similar data were obtained with RAW 264.7 macrophages ( Supplementary Fig. S4b ). Furthermore, the transcript levels of Nos2, Cebpd, Il6, Vegfc and Mmp9 were significantly reduced by ectopic FBXW7α in PPMs ( Fig. 4b ), as was NO production and the glycolytic switch in response to LPS+1% O 2 ( Supplementary Fig. S4c,d ). These data are reminiscent of the phenotype of Cebpd null cells, which express elevated levels of FBXW7α. The profound suppression of LPS-responses by ectopic FBXW7α suggested that upstream elements in the LPS signalling pathway were downregulated by FBXW7α. Intracellular LPS signalling is initiated by TLR4 [1] . Indeed, ectopic FBXW7α reduced expression of TLR4 along with C/EBPδ in PPMs ( Fig. 4c ), while RNAi against Fbxw7α increased the basal and LPS-induced levels of TLR4 and C/EBPδ ( Fig. 4d ). In addition, several pro-inflammatory markers, such as NICD, iNOS and p65, were induced by Fbxw7α -silencing alone ( Fig. 4d ). These data prompted the hypothesis that FBXW7α regulates TLR4 expression through C/EBPδ. The depletion of C/EBPδ prevented the upregulation of TLR4 in response to Fbxw7α silencing ( Fig. 4e ), demonstrating that C/EBPδ mediates TLR4 upregulation. Even basal expression of TLR4 depended on C/EBPδ. Finally, co-expression of degradation-resistant TTS/AAA-C/EBPδ with FBXW7α rescued TLR4 expression in RAW 264.7 macrophages, demonstrating that FBXW7α downregulates TLR4 through the inhibition of C/EBPδ expression ( Fig. 4f ). 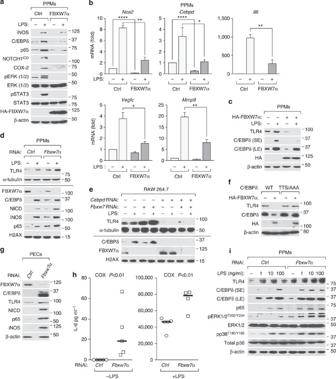Figure 4: FBXW7α suppresses TLR4-mediated LPS responses through C/EBPδ. (a) Western analysis of NE from PPMs transfected with vector or FBXW7α expression constructs and treated with LPS (100 ng ml−1, 16 h) as indicated. (b) RT–qPCR of the indicated mRNA levels in PPMs nucelofected with FBXW7α expression plasmids and treated with LPS (100 ng ml−1, 16 h) as indicated (n=3, *P<0.05, **P<0.001, ****P<0.0001). (c) Western analysis of PPMs transfected with HA-FBXW7α and treated with LPS (100 ng ml−1, 16 h) as indicated. SE, short exposure; LE, long exposure. (d) Western analysis of proteins from PPMs nucleofected with control orFbxw7αsiRNA oligos and treated±LPS (100 ng ml−1, 16 h). The line separates analysis of cytoplasmic (top) and nuclear (bottom) extracts. (e) Western analysis of RAW 264.7 macrophages transfected with siRNA oligos against endogenousCebpdorFbxw7αalone or in combination and treated with LPS (100 ng ml−1, 16 h) as indicated. The line separates analysis of cytoplasmic (top) and nuclear (bottom) extracts. (f) Western analysis of RAW 264.7 macrophages transfected with the indicated expression plasmids. (g) Western analysis of PECs isolated from FVB/N mice 48 h after injection of RNAi againstFbxw7αor control siRNA. (h) Plasma IL-6 concentrations from mice injected with RNAi againstFbxw7α-or control siRNA for 72 h followed by LPS (40 ng) or vehicle (saline) for 1 h. The horizontal line indicates the median IL-6 concentration (n=4–5,Pvalues were determined by the Wilcoxon rank-sum test,P<0.01). (i) Western analysis of PPMs transfected with control orFbxw7αsiRNA oligos and treated with LPS (100 ng ml−1, 4 h) as indicated. SE, short exposure; LE, long exposure. Where applicable, data are mean±s.e.m., evaluated by two-tailed unequal variancet-test (except panel 4 h). Figure 4: FBXW7α suppresses TLR4-mediated LPS responses through C/EBPδ. ( a ) Western analysis of NE from PPMs transfected with vector or FBXW7α expression constructs and treated with LPS (100 ng ml −1 , 16 h) as indicated. ( b ) RT–qPCR of the indicated mRNA levels in PPMs nucelofected with FBXW7α expression plasmids and treated with LPS (100 ng ml −1 , 16 h) as indicated ( n =3, * P <0.05, ** P <0.001, **** P <0.0001). ( c ) Western analysis of PPMs transfected with HA-FBXW7α and treated with LPS (100 ng ml −1 , 16 h) as indicated. SE, short exposure; LE, long exposure. ( d ) Western analysis of proteins from PPMs nucleofected with control or Fbxw7α siRNA oligos and treated±LPS (100 ng ml −1 , 16 h). The line separates analysis of cytoplasmic (top) and nuclear (bottom) extracts. ( e ) Western analysis of RAW 264.7 macrophages transfected with siRNA oligos against endogenous Cebpd or Fbxw7α alone or in combination and treated with LPS (100 ng ml −1 , 16 h) as indicated. The line separates analysis of cytoplasmic (top) and nuclear (bottom) extracts. ( f ) Western analysis of RAW 264.7 macrophages transfected with the indicated expression plasmids. ( g ) Western analysis of PECs isolated from FVB/N mice 48 h after injection of RNAi against Fbxw7α or control siRNA. ( h ) Plasma IL-6 concentrations from mice injected with RNAi against Fbxw7α- or control siRNA for 72 h followed by LPS (40 ng) or vehicle (saline) for 1 h. The horizontal line indicates the median IL-6 concentration ( n =4–5, P values were determined by the Wilcoxon rank-sum test, P <0.01). ( i ) Western analysis of PPMs transfected with control or Fbxw7α siRNA oligos and treated with LPS (100 ng ml −1 , 4 h) as indicated. SE, short exposure; LE, long exposure. Where applicable, data are mean±s.e.m., evaluated by two-tailed unequal variance t -test (except panel 4 h). Full size image FBXW7α suppresses inflammatory signalling Increased basal levels of TLR4 and C/EBPδ protein owing to RNAi against Fbxw7α were also observed in RAW 264.7 macrophages, along with increased transcript levels of the pro-inflammatory genes Cebpd, Tlr4, Tnfa, Il6, Nos2 and Mmp9 in PPMs ( Supplementary Fig. S5a,b ). Taking this approach further, we silenced Fbxw7α in vivo by intraperitoneal injection of small interfering RNA (siRNA). In vivo RNAi can cause non-specific effects that include activation of the immune system [28] . Indeed, control siRNAs led to a modest increase of C/EBPδ expression in PECs compared with vehicle treatment ( Supplementary Fig. S5c ). In comparison, two Fbxw7α RNAi oligos caused a greater increase in both C/EBPδ and TLR4 protein levels. Following this pilot experiment, Ctrl1 and Fbxw7α1 siRNA were used for subsequent analyses. Peritoneal cells that were isolated 2 days after the injection of Fbxw7 α siRNA exhibited reduced FBXW7α levels and higher basal expression of C/EBPδ, TLR4, NICD, p65 and iNOS protein compared with control siRNA ( Fig. 4g ). In addition, transcripts for Cebpd, Nos2 and Il6 were induced ( Supplementary Fig. S5d ). More cells were recovered from Fbxw7 α-siRNA treated mice, indicating the activation of recruitment pathways ( Supplementary Fig. S5e ). However, the ratios of different PECs was not altered ( Supplementary Fig. S5f ). Furthermore, Fbxw7 α siRNA resulted in detectable levels of plasma IL-6 in otherwise untreated mice and in increased IL-6 concentrations in LPS-treated mice ( Fig. 4h ). These data show that endogenous FBXW7α is necessary to prevent pro-inflammatory gene expression. RNAi depletion of FBXW7α in PPMs sensitized the cells, such that 1 ng ml −1 LPS elicited a response that was comparable to 10–100 ng in control cells, as measured by the expression of C/EBPδ and p65 and the phosphorylation of ERK and p38 MAP kinase ( Fig. 4i ). Note that Fbxw7 RNAi increased the basal TLR4 protein levels to LPS-induced levels at this 4 h time point. Taken together, these data show that FBXW7α attenuates the LPS response through inhibition of C/EBPδ and TLR4 expression and that FBXW7α-depletion alone is sufficient to activate inflammatory signalling. TLR4 is a direct transcriptional target of C/EBPδ As C/EBPδ promoted TLR4 protein expression, we next addressed the mechanism underlying this regulation. The loss of C/EBPδ in KO PECs or RNAi-depleted RAW 264.7 macrophages reduced Tlr4 mRNA levels ( Fig. 5a ). Similarly, overexpression of FBXW7α suppressed Tlr4 mRNA levels ( Fig. 5b ), which was consistent with the induced Tlr4 mRNA levels upon Fbxw7α silencing ( Supplementary Fig. S5b ). Interestingly, the expression of Tlr2, Tlr4 and Tlrs 5–9 was also reduced in Cebpd -deficient PPMs, while the expression of Tlr1 and Tlr3 was increased ( Supplementary Fig. S5g ). These data implicate C/EBPδ in the regulation of most Tlr genes. Because of our aforementioned data, we focused our subsequent analyses on TLR4. Inspection of the Tlr4 promoter sequence revealed putative C/EBP-binding sites within 200 bp upstream of the transcription start site ( Fig. 5c ). Chromatin Immunoprecipitation (ChIP) analysis of PPMs demonstrated the binding of C/EBPδ to the proximal Tlr4 promoter region but not to a distal promoter region, where there were no putative binding sites ( Fig. 5c ). Consistent with these data, Cebpd RNAi or FBXW7α overexpression both reduced the activity of a Tlr4 promoter-luciferase reporter construct ( Fig. 5d ). Next, we assessed the effect of TLR4 reconstitution in Cebpd null PPMs ( Fig. 5e ). Overexpression of TLR4 [29] in WT PPMs had no significant effect on the LPS-induced expression of Nos2 and Il6 . In Cebpd -deficient macrophages, however, ectopic TLR4 significantly enhanced LPS-induction of Nos2 and Il6 transcripts ( Fig. 5f ). C/EBPδ binds the Il6 promoter [10] and may regulate the iNOS promoter directly [30] . Our data show that the impaired LPS response of Il6 and Nos2 in Cebpd null macrophages is in part due to reduced TLR4 levels, and it is less owing to the role of C/EBPδ as a downstream effector of TLR4. The role of basal C/EBPδ expression was further supported by an analysis of early LPS signalling events. The accumulation of p65 and the phosphorylation of ERK, p38 and JNK kinases in response to LPS were attenuated in Cebpd null PPMs within 30–60 min of treatment ( Fig. 5g ). In summary, these results show that C/EBPδ also functions upstream of LPS signalling through activation of Tlr4 gene expression. 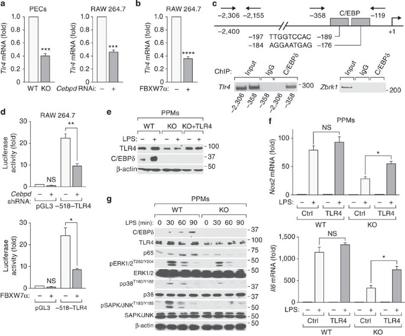Figure 5: TLR4 is a direct transcriptional target of C/EBPδ. (a) RT–qPCR analysis ofTlr4mRNA levels in WT orCebpdKO PECs and in RAW 264.7 macrophages afterCebpdsilencing (n=3, ***P<0.001). (b) RT–qPCR analysis ofTlr4in RAW 264.7 macrophages with or without ectopic FBXW7α (n=3, ****P<0.0001). (c) Schematic of theTlr4promoter with location of putative C/EBP binding sites and of primers used for ChIP. ChIP analysis from PPMs for binding of C/EBPδ to the indicatedTlr4promoter regions. IgG and aZbrk1promoter region served as negative controls. Numbers indicate the position of molecular size markers in base pairs. (d) Luciferase reporter assay in RAW 264.7 macrophages transfected with the indicated luciferase reporter and shRNA againstCebpd(top panel) or FBXW7α expression constructs (bottom panel) (n=3, *P<0.05, **P<0.001). NS, not significant. (e) Western analysis of PPMs from WT andCebpdKO mice transfected with TLR4 expression plasmids as indicated. (f) RT–qPCR analysis of the indicated mRNA levels in PPMs as in panel (e). (n=3, *P<0.05; NS, not significant). (g) Western analysis of PPMs from WT andCebpdKO mice treated with 200 ng ml−1LPS for the indicated times. Where applicable, data are mean±s.e.m., evaluated by two-tailed unequal variancet-test. Figure 5: TLR4 is a direct transcriptional target of C/EBPδ. ( a ) RT–qPCR analysis of Tlr4 mRNA levels in WT or Cebpd KO PECs and in RAW 264.7 macrophages after Cebpd silencing ( n =3, *** P <0.001). ( b ) RT–qPCR analysis of Tlr4 in RAW 264.7 macrophages with or without ectopic FBXW7α ( n =3, **** P <0.0001). ( c ) Schematic of the Tlr4 promoter with location of putative C/EBP binding sites and of primers used for ChIP. ChIP analysis from PPMs for binding of C/EBPδ to the indicated Tlr4 promoter regions. IgG and a Zbrk1 promoter region served as negative controls. Numbers indicate the position of molecular size markers in base pairs. ( d ) Luciferase reporter assay in RAW 264.7 macrophages transfected with the indicated luciferase reporter and shRNA against Cebpd (top panel) or FBXW7α expression constructs (bottom panel) ( n =3, * P <0.05, ** P <0.001). NS, not significant. ( e ) Western analysis of PPMs from WT and Cebpd KO mice transfected with TLR4 expression plasmids as indicated. ( f ) RT–qPCR analysis of the indicated mRNA levels in PPMs as in panel ( e ). ( n =3, * P <0.05; NS, not significant). ( g ) Western analysis of PPMs from WT and Cebpd KO mice treated with 200 ng ml −1 LPS for the indicated times. Where applicable, data are mean±s.e.m., evaluated by two-tailed unequal variance t -test. Full size image C/EBPδ augments inflammatory signalling in tumours TLR4 is expressed in both macrophages and tumour cells [4] . Proteins such as HMGB1 and S100A8 act as ligands that activate TLR4 signalling, and these ligands are important in tissue repair, inflammatory diseases and cancer [3] , [31] , [32] . Inflammation-associated gene expression is strongly correlated with tumour malignancy [33] . Given that C/EBPδ promotes metastatic progression of MMTV-Neu mammary tumours [13] , we investigated whether C/EBPδ modulates TLR4 expression in tumour cells. Stable depletion of C/EBPδ in a mouse mammary tumour cell line or in human MCF-7 breast tumour cells reduced TLR4 protein expression and induced FBXW7α levels ( Fig. 6a ). Analyses of MMTV-Neu tumour tissue confirmed the reduced Tlr4 mRNA, increased Fbxw7 mRNA, and, on average, lower TLR4 protein levels in Cebpd −/− tumours compared with WT ( Fig. 6b ). In addition, iNOS protein expression ( Fig. 6b ) and Il6, Nos2, Arg1 and Tnfa transcript levels were lower in Cebpd −/− tumours ( Fig. 6c ). Interestingly, the transcript levels of Il10 and Il13 , which are expressed in cells including alternatively activated macrophages and T cells, were significantly higher in Cebpd −/− tumours ( Fig. 6c ). The inverse correlation of Cebpd and Il10 expression in vivo is consistent with a previous report on C/EBPδ functions in dendritic cells [12] . 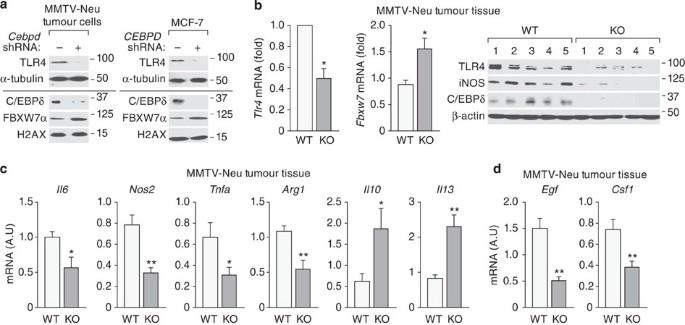Figure 6:Cebpd nulltumours exhibit reduced expression of TLR4 and altered expression of inflammatory genes. (a) Western analysis of proteins from an MMTV-Neu tumour cell line or MCF-7 cells with stable shRNA-silencing of C/EBPδ expression or control shRNA. The line separates analysis of cytoplasmic (top) and nuclear (bottom) extracts. (b) RT–qPCR analysis ofTlr4andFbxw7mRNA (left panels) and Western analysis (right panel) of protein from MMTV-Neu tumours of WT andCebpdKO mice (n=5, *P<0.05). (c,d) RT–qPCR analysis of mRNA levels of the indicated genes in MMTV-Neu tumour tissue from WT andCebpdKO mice. A.U., arbitrary units. (n=6, *P<0.05; **P<0.001). Where applicable, data are mean±s.e.m., evaluated by two-tailed unequal variancet-test. Figure 6: Cebpd null tumours exhibit reduced expression of TLR4 and altered expression of inflammatory genes. ( a ) Western analysis of proteins from an MMTV-Neu tumour cell line or MCF-7 cells with stable shRNA-silencing of C/EBPδ expression or control shRNA. The line separates analysis of cytoplasmic (top) and nuclear (bottom) extracts. ( b ) RT–qPCR analysis of Tlr4 and Fbxw7 mRNA (left panels) and Western analysis (right panel) of protein from MMTV-Neu tumours of WT and Cebpd KO mice ( n =5, * P <0.05). ( c , d ) RT–qPCR analysis of mRNA levels of the indicated genes in MMTV-Neu tumour tissue from WT and Cebpd KO mice. A.U., arbitrary units. ( n =6, * P <0.05; ** P <0.001). Where applicable, data are mean±s.e.m., evaluated by two-tailed unequal variance t -test. Full size image We also examined the expression of chemokines and chemokine receptors, which have an important role in breast tumour progression and metastasis [34] . C ebpd KO tumours exhibited significantly reduced expression of the metastasis-promoting gene Cxcr4 , which was consistent with our previous report that C/EBPδ directly regulates Cxcr4 in cultured mammary tumour cells [5] . In contrast, C/EBPδ-null tumours exhibited increased expression of Ccl3 and Ccl5 , which augment T-cell mediated anti-immune responses [35] ( Supplementary Fig. S6 ). Of these genes, the Ccl3 gene promoter is directly bound by C/EBPδ after LPS induction [4] . Collectively, these data show that the loss of C/EBPδ leads to complex alterations of pro-and anti-inflammatory genes in mammary tumour tissue and that this complexity may be owing to its multifaceted roles in macrophages and mammary epithelial cells. Macrophages and tumour cells engage in crosstalk, and a metastasis-promoting paracrine loop has been described with breast carcinoma cells producing colony stimulating factor-1 (Csf1) and macrophages expressing epidermal growth factor (EGF) [36] . We found that both Csf1 and Egf expressions were significantly reduced in Cebpd null MMTV-Neu mammary tumours ( Fig. 6d ). Though further analyses will be required to dissect the contribution of different cell types to these observations, the results are likely due to C/EBPδ action in both the immune cells and tumour cells. In summary, these data show that C/EBPδ activity profoundly affects the expression of proteins that are modulators of the immune system, which collectively creates a largely pro-inflammatory microenvironment in mammary tumours. In this study, we identified a positive feedback loop between C/EBPδ and TLR4 and a negative feedback loop between C/EBPδ and FBXW7α, which together modulate TLR4 signalling and pro-inflammatory gene expression ( Fig. 7 ). Phosphorylation of C/EBPδ by GSK-3β is required for its degradation by FBXW7α. Therefore, inhibition of GSK-3β by LPS stabilizes C/EBPδ. Identification of TLR4 as a direct transcriptional target of C/EBPδ renders C/EBPδ a pro-inflammatory factor upstream of TLR4 in addition to its functions downstream. 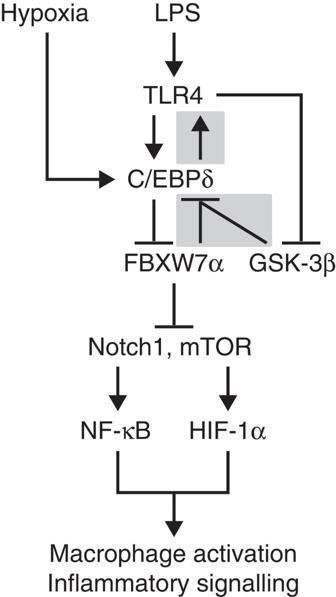Figure 7: Schematic describing the feedback loops between TLR4, C/EBPδ and FBXW7α that control LPS signalling. The shaded boxes indicate the elements of this pathway that were identified in this study. Figure 7: Schematic describing the feedback loops between TLR4, C/EBPδ and FBXW7α that control LPS signalling. The shaded boxes indicate the elements of this pathway that were identified in this study. Full size image Macrophages can be activated by several pathways, and C/EBPδ together with C/EBPβ also participates in Fcγ receptor-mediated inflammatory cytokine and chemokine production and in IgG IC-stimulation of macrophages [37] . In addition to our data, the regulation of Tlr8 expression by C/EBPδ as well as its binding to the Tlr6 gene promoter have been reported [10] , [38] . A critical role of C/EBPδ in LPS responses has previously been shown in vitro and in vivo . Cebpd null mice are hypersensitive to persistent bacterial infection [10] and hyposensitive to septic shock after sensitization [11] . Both phenotypes were attributed to the role of C/EBPδ as an inflammatory response gene and regulator of target genes such as Il6 . Furthermore, the role of C/EBPδ in amplifying LPS signalling has been described [39] . It should be noted that one study reported that C/EBPδ is dispensable for LPS-induced Il6 expression [40] . It remains to be determined which experimental details are responsible for the difference in results. Our findings place C/EBPδ upstream of LPS signalling for expression of the TLR4 receptor. The loss of C/EBPδ does not abolish Tlr4 expression entirely, which explains why LPS responses are not completely impaired. Interestingly, our data from reconstituting Cebpd −/− cells with ectopic TLR4 suggest that the precise role of C/EBPδ downstream of TLR signalling should be re-evaluated in light of its role in regulating TLR4 expression. Low dose LPS specifically induces C/EBPδ expression rather than NF-kB [41] , supporting the notion that C/EBPδ is critical in sensitizing cells to LPS. Our data show that C/EBPδ promotes macrophage activation in part by augmenting HIF-1α expression. Inflamed tissue is hypoxic and HIF-1 mediates hypoxia adaptation by regulating the transcription of many genes associated with angiogenesis, glycolysis and migration [16] . C/EBPδ also promotes tumour lymphangiogenesis through HIF-1 [42] . Our results show that macrophage functions that require HIF-1 are blunted in the absence of C/EBPδ because of Fbxw7α derepression. HIF-1α expression in the myeloid lineage also promotes the differentiation of myeloid-derived tumour suppressor cells, which contribute to tumour progression [17] , [18] , [43] . This mechanism may underlie the pro-metastatic function of C/EBPδ in addition to the role of this pathway in epithelial-derived tumour cells [13] . Interestingly, TLR4 is also a target of HIF-1 (ref. 44 ); hence, C/EBPδ induces TLR4 expression directly under normoxia and also indirectly through HIF-1 induction under hypoxia. This effect provides an additional positive feedback loop because C/EBPδ is a hypoxia-induced gene that is likely downstream of HIF-1 (refs 13 , 42 ). However, this pro-inflammatory loop requires simultaneous inhibition of FBXW7α expression by C/EBPδ, suggesting that FBXW7α serves as an important brake on inflammatory signalling. In this study, we found that Cebpd -deficient mouse mammary tumour tissues, which exhibit reduced metastatic progression [13] , express increased FBXW7α and reduced TLR4 levels. The effects of TLR4 signalling on cancer appear complex and may depend not only on the cell type but also on the stage of tumour development [6] , [7] , [45] , [46] , [47] , [48] . In our study, reduced TLR4 expression in Cebpd null tumours correlated with mostly reduced pro-inflammatory and increased anti-inflammatory gene expression. This result may be due to the role of C/EBPδ in mammary tumour cells and infiltrating immune cells, direct targeting by C/EBPδ, or indirect downstream effects. Interestingly, reduced innate immune responses in Cebpd null mice are also consistent with the increased mammary tumour multiplicity in these mice [13] . Our data warrant further dissection of the role of C/EBPδ in tumour-associated macrophages and their crosstalk with mammary tumour cells, which will be addressed by conditional gene deletion in future analyses. From this study, FBXW7α emerged as a potent attenuator of inflammatory signalling. This activity is at least in part due to suppression of C/EBPδ expression at the protein and mRNA levels and is likely to affect not only Cebpd but also other genes/proteins that modulate inflammation. Therefore, our data lay the groundwork for further analyses of FBXW7α functions in the modulation of immune cells. We also suggest that the tumour suppressor activity of FBXW7 [14] could be in part due to its role as an attenuator of pro-inflammatory gene expression. According to the ‘1000 Genomes’ catalogue ( www.1000genomes.org ), the FBXW7 gene harbours several SNPs, some with possibly deleterious effects on function. We suggest that these SNPs be included in genome-wide association studies of inflammatory diseases. Given the role of FBXW7α as a suppressor of inflammatory signalling (as shown in this study) and as a bona fide tumour suppressor [14] , [15] , FBXW7α is an unlikely therapeutic target. However, better knowledge of the regulation of its expression and its target proteins may provide new avenues for the management of inflammation-associated diseases. Reagents and antibodies LPS (from E. coli ; L4524) was purchased from Sigma-Aldrich, St Louis, MO. CHIR99021 and BIO (6-Bromoindirubin-3′-oxime) were obtained from Stemgent, San Diego, CA. Antibodies were obtained from the following sources: Cell Signaling Technology (pGSK-3β-Ser9, no. 9336; pAKT-Ser473, no. 4060; pS6K1-Thr389, no. 9205; pSTAT3, no. 9145; AKT, no. 4691; GSK-3β, no. 9315; S6K1, no. 9202; STAT3, no. 4904; Cleaved Notch-1, no. 2421S; phospho-p44/42 MAPK-Thr202/Tyr204 (pErk1/2), no. 9101; p44/42 MAPK (Erk1/2), no. 9102; pp38-Thr180/Tyr182, no. 9215S; p38, no. 9212; pSAPK/JNK-Thr183/Tyr185, no. 4668S; SAPK/JNK, no. 9258; phospho-threonine, no. 9386S); Abcam (iNOS, no. ab-15323; F4/F80, no. ab-60343-100; Cox-2, no. ab-15191; p65 (RelA); no. ab-16502; FBXW7, ab no. 12292); BD Pharmingen (CD11b (M1/70), no. 550993; GR1, no. 553128; CD16/CD32, no. 553142); Novus Biologicals (HIF-1α, no. NB100-449; HIF-1β, no. NB-100-124); Santa Cruz (actin, sc-1616; Ubiquitin, sc-8017); Calbiochem (mTOR, no. OP97); Orbigen (FBXW7alpha, no. PAB-10563); BD Biosciences (Aurora A, no. 610938); Imgenex (TLR4, no. IMG-578A); Bethyl Laboratories (H2AX, no. A300-083A); eBioscience (B220, no. RA3-6B2; CD3e, no. 500A-2, and isotype controls); Roche (HA, no. 11867423001; clone3F10); and Rockland (Tubulin, no. 600-401-880). The mouse monoclonal antibody clone L46-743.92.69 (batch BD69319) against C/EBPδ was provided by BD Biosciences Pharmingen as an outcome of an Antibody Co-development Collaboration with the NCI. For information on plasmids see Supplementary Methods . Mice and isolation of peritoneal cells Cebpd wild-type and knockout mice [49] were of the FVB/N strain background (except for data in Supplementary Fig. S2 , which are from 129S1 mice) and derived from heterozygous mates. The MMTV-c-Neu tumour model has been described [13] , [19] . The subjects were littermates whenever possible. NCI-Frederick (FNLCR) is accredited by AAALLC International and follows the Public Health Service Policy for the care and use of laboratory animals. All experiments were conducted according to protocols approved by the Institutional Animal Care and Use Committee. For the isolation of PPMs, mice were injected with 3% Brewer thioglycollate medium [50] in the peritoneal cavity. Four days later, mice were killed, and 10 ml sterile PBS (Ca 2+ /Mg 2+ -free) was injected into the peritoneal cavity. The resulting peritoneal fluid was collected and centrifuged at 400 g for 10 min at 4 °C. The cell pellet was washed once with PBS. Erythrocytes were lysed with sterile water, and the final pellet was suspended in 1:1 DMEM/F12 medium with 10% foetal bovine serum (FBS). Viability was >95%. Cell preparations were characterized by FACS analysis using antibodies that distinguish macrophages from other hematopoietic cells. On average, 82.5±3.7% (mean±s.e.m., n =6) of the cells were Mac-1 + and F4/80 + before plating. The isolated cells were plated and allowed to adhere for 2 h. Non-adherent cells were washed off with PBS, and new culture medium was added. Cells were cultured for 24 h before experimental treatments. Resident PECs were isolated as described above but without prior elicitation by thioglycollate. For details, see Supplementary Methods . Cell culture MMTV-Neu and MCF-7 cell lines with stable depletion of C/EBPδ were generated by transfection of expression constructs for shRNA against C/EBPδ (or green fluorescent protein (GFP) as a control [13] ). Cells were selected in G418 and maintained as pools. ANA-1, RAW 264.7 mouse macrophages and HEK293T cells were cultured in DMEM containing 10% FBS. PPMs and PECs were cultured in DMEM/F12 medium containing 10% FBS. The U-937 human monocytic cell line and elutriated primary human monocytes were cultured in RPMI medium containing 5% FBS. The MMTV-Neu mouse mammary tumour cell line (a kind gift of Dr William Muller, McGill University) was cultured in DMEM containing 5% FBS and 1X-MEGS (mammary epithelial cell growth supplement). Unless indicated otherwise, LPS was used at 100 ng ml −1 for 16–24 h. Peripheral blood-derived monocytes were isolated from healthy donors by counterflow centrifugal elutriation under protocols approved by the Institutional Review Boards of both the National Institute of Allergy and Infectious Diseases and the Department of Transfusion Medicine of the National Institutes of Health after appropriate informed consent. Transient transfections and RNAi Cells were transfected by nucleofection using the Amaxa Cell-line Nucleofector Kit V (Cat no. VCA-1003; Lonza AG). A GFP expression construct was included in all transfections to monitor transfection efficiency. The total amount of DNA in each transfection was kept constant by complementation with vector control DNA. All control samples were transfected with vector only. At 24 h post-transfection, cells were treated as indicated. Cebpd siRNA oligos were purchased from Dharmacon (no. L-003210-00). Fbxw7-specific siRNAs (Silencer predesigned) with the following sequences were used [13] , [51] . Fbxw7α RNAi-1: 5′-GGGCAGCAGCGGCGGAGGAdTdT-3′ and antisense: 5′-UCCUCCGCCGCUGCUGCCCdTdT-3′. Fbxw7α RNAi-2: Sense: 5′-GCACAGAAAAUUGAUACAACTT-3′ and antisense: 5′-GUUAGUAUCAAUUCUGUGCTG-3′ Fbxw7α RNAi-3: 5′-GUGAAGUUGUUGGAGUAGAdTdT-3′ and antisense: 5′-UCUACUCCAACAACUUCACdTdT-3′. Fbxw7 RNAi-4: Sense: 5′-GCACAGAAUUGAUACAACTT-3′ and antisense: 5′-GUUAGUAUCAAUUCUGUGCTG-3′. For silencing Fbxw7α in mouse cells, Fbxw7α RNAi-1 ( in vitro and in vivo ) and RNAi -2 ( in vivo ) were used. Fbxw7α RNAi-3 and Fbxw7 RNAi-4 were used at a 1:1 ratio in human cells. Scrambled siRNA (no. D-001960-01-05, Dharmacon) or EGFP siRNA [51] (5′-CAAGCTGACCCTGAAGTTC-3′) were used as controls. For in vivo RNAi, mice were injected in the peritoneum with in vivo- jetPEI (Polyplus) according to the manufacturer’s instructions. For details see Supplementary Methods . Western analysis and In vitro ubiquitination assay See Supplementary Methods Pulse-chase experiment RAW264.7 cells were transfected with control or Fbxw7α siRNA oligonucleotides. Two days later, the cells were pre-incubated for 30 min in DMEM without methionine and cysteine, pulsed with Tran 35 S-label (ICN; 300 μCi ml −1 ; 1 μCi=37 kBq) for 20 min, and chased with DMEM/10% FBS plus 20 mM methionine and cysteine for the indicated times. Cells were lysed under denaturing conditions, and proteins were immunoprecipitated with anti-CEBPδ antibody and protein G beads. After SDS-PAGE, the dried gel was processed for phosphorimaging. Signals were quantified by ImageQuant software and plotted using GraphPad Prism 5. Plasma IL-6 measurement FVB/N mice were injected intraperitoneally with control or Fbxw7α siRNA (100 μg) using in vivo- jetPEI (Polyplus) according to the manufacturer’s instructions. Three days later, mice were injected with LPS (40 ng) or vehicle (saline) and killed 1 h later to collect heparinized blood. IL-6 was measured in plasma using a mouse IL-6 single analyte ELISA kit according to the manufacturer’s instructions (SA Biosciences, Qiagen, USA, no. SEM03015A). RNA isolation and quantitative real-time PCR RNA was isolated using TRIZOL (Invitrogen), and cDNA was synthesized with Superscript reverse transcriptase III (RT) according to the manufacturer’s instructions (Invitrogen, CA). PCR was performed with Taqman gene expression primer/probe sets using the 7500 Fast Real-Time PCR instrument (Applied Biosystems). Analysis was performed using the MxPro Software (Stratagene). All reactions were performed in duplicates with ‘no RT’ as the control, and all data are mean±s.e.m. of at least three independent biological replicates. The relative expression levels were measured using the relative quantitation ΔΔCt method and normalized to β-actin. The probe sets (Applied Biosystems) were as follows: Cebpd : Mm00786711_s1; Fbxw7a : Mm01209394_m1; Tlr4 : Mm00445273_m1; Il6 : Mm59999064_m1; Mmp9 : Mm00442991_m1; Cxcr4 : Mm01292123_m1; Vegfc : Mm01202432; Nos2 : Mm00440502; Tnfa : Mm00443258_m1; Il10 : Mm00439614_m1; Arg1 : Mm00475988_m1; Il13 : Mm00434204_m1; mCsf-1 : Mm00432686_m1; Egf ; Mm01316968_m1; Ccl3 ; Mm00441259_g1; Ccl5 : Mm01302427_m1; Actin : 4352933-0711018. Chromatin Immunoprecipitation assay ChIP analysis was performed per the manufacturer’s instructions (EZ ChIP, no. 17-371 RF, Millipore, USA). PPMs at 80–90% confluency were cross-linked, and the chromatin was prepared and sonicated to an average size of 500 bp. The DNA fragments were immunoprecipitated with antibodies specific to C/EBPδ (5 μg; BD69319) or control mouse IgG at 4 °C overnight. RAW 264.7 macrophages were nucleofected with control or Fbxw7 siRNA oligos. Forty-eight hours later, cells were processed as above. After reversal of the cross-linking, the immunoprecipitated chromatin was amplified by PCR as follows: Tlr4 , 1 cycle of 94 °C 3 min, 35 cycles of 94 °C 20 s, 56 °C 30 s, and 72 °C 30 s, and 1 cycle of 72 °C 2 min; Zbrk1 , 1 cycle of 94 °C 3 min, 37 cycles of 94 °C 20 s, 56 °C 30 s and 72 °C 30 s, and 1 cycle of 72 °C 2 min. Cebpd, 1 cycle of 94 °C 3 min, 40 cycles of 94 °C 20 s, 56 °C 30 s, and 72 °C 30 s, and 1 cycle of 72 °C 2 min. The primers were as follows: Tlr4 proximal: Tlr4-(S): 5′-ACAAGACACGGCAACTGATG-3′ Tlr4-(AS): 5′-GCTTTCATCCCAGGAAGTCA-3′ Tlr4 distal: Tlr4-(S): 5′-GCCAAGAAGCTCCACAGAG-3′ Tlr4-(AS): 5′-CATCACTAGTCCAGTCGATACCC-3′ Cebpd: Cebpd- (S): 5′-TGATCCCTGTTCCGCCTTTGCTAT-3′ Cebpd- (AS): 5′-AGTGGGTCGGAGACCGGA-3′ Zbrk1 : Zbrk1-(S): 5′-CATTCTCTGGGATACCTACACCTG-3′ Zbrk1(AS): 5′-CTGTAAAATGGCCGCGCCCATAGC-3′ In vitro kinase assay For in vitro phosphorylation analysis, C/EBPδ was immunoprecipitated with anti-C/EBPδ antibody from radioimmunoprecipitation assay buffer extracts of HEK293T cells transfected with WT or TTS/AAA C/EBPδ and incubated with 100 ng recombinant GSK-3β in kinase assay buffer, as described previously [52] . Samples were resolved on SDS-PAGE gels and subjected to autoradiography. The labelled C/EBPδ proteins were digested from the gel with pepsin and analysed by reverse-phase high-performance liquid chromatography, phosphoamino acid analysis and Edman degradation [52] . Luciferase reporter assay RAW 264.7 cells were transfected with TLR4 promoter luciferase reporter constructs [53] , renilla luciferase expression plasmids along with the indicated expression constructs. To silence C/EBPδ expression, two different short hairpin RNA expression constructs were used at 1:1 ratio, and shRNA against GFP was used as control [13] . Forty-eight hours later, luciferase activity was assessed using a luciferase assay kit according to manufacturer’s instructions (Promega). Metabolic measurements Measurements of lactate, glucose, ATP and NO were as described in Supplementary Methods . Statistical analysis Unless stated otherwise, quantitative data were analysed by the two-tailed unequal variance t -test and are shown as the mean±s.e.m. The number of samples (n) refers to biological replicates. How to cite this article: Balamurugan, K. et al . FBXW7α attenuates inflammatory signalling by downregulating C/EBPδ and its target gene Tlr4 . Nat. Commun. 4:1662 doi: 10.1038/ncomms2677 (2013).